Design ofC1-symmetric tridentate ligands for enantioselective dearomative [3 + 2] annulation of indoles with aminocyclopropanes Chiral polycyclic indolines are widely present in natural products and have become the focus of extensive synthetic efforts. Here, we show the catalytic asymmetric dearomative [3 + 2] annulation of indoles with donor-acceptor aminocyclopropanes to construct tricyclic indolines. Key to the success of the reaction is the rational design of C 1 -symmetric bifunctional tridentate imidazoline-pyrroloimidazolone pyridine ligand. Under 5 mol% of Ni(OTf) 2 -ligand complex, diverse tricyclic indolines containing cyclopentamine moieties are obtained in good chemoselectivities, high diastereoselectivities, and excellent enantioselectivities. An unusual cis -configuration ligand is superior to the trans -configuration ligand and the corresponding C 2 -symmetric tridentate nitrogen ligands in the annulation reaction. Mechanistic studies by control experiments and density functional theory calculations reveal a dual activation manner, where Ni(II) complex activates the aminocyclopropane via coordination with the geminal diester, and imidazolidine NH forms a H-bond with the succinimide moiety. Chiral polycyclic indolines exist widely in natural products, which often contain cyclic amine fragments, such as vindolinine [1] , N -methylkopsanone [2] , and vincadifformine [3] (Fig. 1a ). For their construction, catalytic asymmetric dearomatization (CADA) reaction of indoles is a powerful strategy [4] , [5] , [6] , [7] , [8] , [9] , [10] , [11] . In 2013, Tang and co-workers pioneered the highly enantioselective cyclopentannulation of indoles with donor–acceptor (D-A) aryl cyclopropanes catalyzed by a chiral side armed bisoxazoline (SaBox)-Cu(OTf) 2 complex [12] , [13] , [14] , [15] , [16] , [17] . Later, Waser and co-workers reported the catalyzed reaction of D-A aminocyclopropanes with C3-substituted indoles, producing C2-alkylated products instead of [3 + 2] annulation products (Fig. 1b ) [18] . In 2019, Wang and co-workers developed Rh(II) carbene triggered cyclopentannulation reaction to form diverse polycyclic indolines with high yields, in which D-A aminocyclopropanes were formed in situ (Fig. 1c ) [19] . In 2021, Waser and co-workers described the catalytic [3 + 2] annulation of D-A aminocyclopropane monoesters and indoles in high yields and diastereoselectivities catalyzed by triethylsilyl triflimide [20] . In order to construct chiral tricyclic indolines containing cyclopentamine moieties, we envisaged the utilization of the catalytic asymmetric dearomative [3 + 2] annulation reaction of D-A aminocyclopropanes with C3-substituted indoles. However, this approach possesses some challenges related to chemo-, diastereo-, and enantioselectivity (Fig. 1d ). Fig. 1: Significances and reactions of D-A cyclopropanes with substituted indoles. a Chiral polycyclic indolines containing cyclic amine fragments in natural products. b Previous work: the reaction of D-A aminocyclopropanes with C3-substituted indoles produces C2-alkylated product from Waser et al. c Previous work: Rh(II) carbene triggered cyclopentannulation reaction of in situ formed D-A aminoacyclpropanes from Wang et al. d This work: catalytic asymmetric dearomative [3 + 2] annulation reaction of D-A aminocyclopropanes with C3-substituted indoles. D-A donor–acceptor. Full size image The design and development efficient chiral tridentate nitrogen ligands bearing a pyridine ring is an attractive goal in asymmetric catalysis [21] , [22] , [23] , [24] , [25] , [26] , [27] , [28] . C 1 -Symmetric tridentate nitrogen ligands have the ability to connect two different chiral moieties, hence, exhibit a greater capacity for structural tuning. Notable C 1 -symmetric tridentate nitrogen ligands include pyridyl-based benzimidazolyl-oxazolyl ligand [29] , bis(imino)pyridine [30] , iminopyridine-oxazoline (IPO) [31] , [32] , oxazoline aminoisopropylpyridine (OAP), imidazoline iminopyridine (IIP) and thiazoline iminopyridine (TIP) [33] . In 2010, Arai and co-workers developed bis(imidazolidine)pyridine (PyBidine) as a highly efficient bifunctional tridentate nitrogen ligand with imidazolidine NH as H-bond donor, and proved that imidazolidine was a privileged chiral moiety [34] , [35] . Recently, in 2022, our group reported bis(pyrroloimidazolone)pyridine (PyBPI) as a bifunctional tridentate ligand, in which pyrroloimidazolone framework [36] , [37] formed a non-flat chiral fence [38] . By incorporating imidazoine and pyrroloimidazolone into the pyridine skeleton, we designed a C 1 -symmetric tridentate imidazoline-pyrroloimidazolone pyridine (PyIPI) ligands (Fig. 2a ). Fig. 2: Design, synthesis, and application of PyIPI ligands. a Design and synthesis of PyIPI ligands. b X-ray structure of Cu(OTf) 2 -PyIPI L1 complex. c Metal-PyIPI complex catalyzed asymmetric dearomative [3 + 2] annulation of indoles with donor–acceptor aminocyclopropane. PyIPI imidazoline-pyrroloimidazolone pyridine. Full size image PyIPI ligand was facilely synthesized from pyridine-2,6-dicarbaldehyde in twice condensation reactions with L-prolinamide and ( R , R )-diphenylethylenediamine, respectively. PyIPI ligand readily formed a metal complex with Cu(OTf) 2 , which was determined by X-ray diffraction analysis of a single crystal (Fig. 2b ). The central Cu metal displayed a pentacoordinated square pyramidal geometry, where three nitrogen atoms and two triflate ligands were bonded to the central metal. Furthermore, H-bonding existed between the imidazolidine NH atom and one oxygen atom of triflate anion, with a distance of 2.439 Å. We hypothesized that PyIPI may exhibit the following features: (1) the tridentate nitrogen ligand could coordinate with different Lewis acids, and imidazolidine NH could act as H-bond donor, thus playing a bifunctional role; (2) the bicyclic pyrroloimidazolone moiety formed a non-flat chiral fence, and exerted an enhanced steric hindrance effect; (3) the configuration of newly formed sp 3 carbons was tunable, resulting in greater catalyst variability; (4) the steric hindrance of two amine moieties could remotely control the chiral environment created by a tridentate nitrogen ligand; (5) the two different chiral sources were cheap and readily available. In this work, we envisage that PyIPI coordinates with a metal to activate the aminocyclopropane via bidentate coordination with two carbonyl oxygen atoms, and imidazolidine NH forms a H-bond with the oxygen atom in succinimide moiety, thus resulting in a dual activation and creating a good stereocontrol in [3 + 2] annulation with indoles (Fig. 2c ). 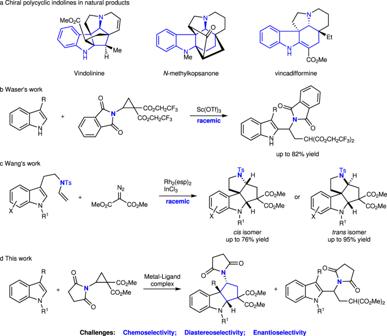Fig. 1: Significances and reactions of D-A cyclopropanes with substituted indoles. aChiral polycyclic indolines containing cyclic amine fragments in natural products.bPrevious work: the reaction of D-A aminocyclopropanes with C3-substituted indoles produces C2-alkylated product from Waser et al.cPrevious work: Rh(II) carbene triggered cyclopentannulation reaction of in situ formed D-A aminoacyclpropanes from Wang et al.dThis work: catalytic asymmetric dearomative [3 + 2] annulation reaction of D-A aminocyclopropanes with C3-substituted indoles. D-A donor–acceptor. Optimization study Initially, the reaction of indole 1a with racemic succinimido-substituted dimethyl ester cyclopropane 2a was selected as the model reaction under PyIPI L1 as the chiral ligand in CH 2 Cl 2 at 25 °C (Table 1 ). When Cu(OTf) 2 was used as the central metal salt, the reaction proceeded in low yield, affording a mixture of tricyclic indoline 3a and C2 alkylation product 4a in a ratio of 83:17, in which major product 3a had 7:1 diastereoselectivity and 81% ee (entry 1). Hence, several metal salts were evaluated (entries 2-8), where Ni(OTf) 2 showed the best results (91% total yield, 3a / 4a = 80:20, 8:1 dr, and 83% ee, entry 7). In the case of PyIPI L2 , derived from trans -4-hydroxyl-L-prolinamide, low ee of 3a was observed (entry 9). Chiral PyIPI L3 ‒ L6 that contained different sterically hindered amide substituents were tested (entries 10–13). PyIPI L4 , bearing a phenyl group on aniline, exhibited higher catalytic activity and enhanced stereocontrol (entry 11). Hence, PyIPI L4 was used as the ligand to examine different nickel salts such as Ni(BF 4 ) 2 ∙6H 2 O, Ni(ClO 4 ) 2 ∙6H 2 O, and Ni(OAc) 2 . However, the obtained results did not show any enhancement (Supplementary Table 1 ). ( S , S )-Diphenylethylenediamine derived PyIPI L7 with a common trans -configuration was employed, resulting in a dramatic decrease in ee value of product 3a (entry 14), indicating the importance of the unusual cis -configuration in L4 . Utilization of C 2 -symmetric tridentate nitrogen ligands L8 and L9 showed low catalytic activity and poor ee values (entries 15 and 16), which illustrated the significance of C 1 -symmetry in L4 . Increasing the ratio of aminocyclopropane 2a to 2.2 equiv., further improved ee value of 3a with 98% ee (entry 17). Altering the catalytic loading demonstrated that 5 mol% of Ni(OTf) 2 - L4 complex was optimal; however, even 2.5 mol% of catalyst still afforded product 3a in 95% ee (entries 18 and 19). In comparison, other commonly used chiral ligands, such as chiral bisoxazoline (Box) and pyridine-bisoxazoline (Pybox) were also tested. However, with t Bu-Box or t Bu-Pybox as ligands and Ni(OTf) 2 as the central metal, the reaction did not happen under the same conditions (entries 20 and 21). Table 1 Optimization of the reaction conditions a Full size table Scope of the reaction Under optimal reaction conditions (Table 1 , entry 18), the substrate scope of the asymmetric dearomative [3 + 2] annulation was explored (Fig. 3 ). Compared with 5-methyl- and 5-methoxy-substituted indoles 1b and 1c , the reaction of 5-chloro- and 5-bromo-substituted indoles 1d and 1e were slower, while the influence of electronic effect on enantioselectivity was negligible ( 3b – 3e ). 6-Bromo-substituted indole 1f afforded annulation product 3f in satisfactory results. C3-Allyl-substituted indole 1g and C3-alkoxy-substituted indoles 1h - i also proceeded smoothly, delivering tricyclic indoline 3g-i in good results with 93–97% ee. In the case of penta-fused indole 1j , [3,3,3,0]-tetracyclic indoline 3j was obtained in 96% ee, albeit with low diastereoselectivity. Meanwhile, the reaction of 1,2,3-trimethylindole 1k also proceeded well, delivering indoline 3k in 65% yield, 4:1 dr, and 97% ee. It should be pointed out that indoles without a C3 substituent usually afforded only the products of Friedel-Crafts at C3 position, rather than the expected [3 + 2] annulation products (Supplementary Fig. 5 ). N -Benzyl indole 1l gave [3 + 2] annulation product 3l in good results. With 3-phenylindole 1m as the reactant, the [3 + 2] annulation reaction could be occurred with Cu(OTf) 2 - L4 as the catalyst, affording the tricyclic product 3m in 51% yield, 1.8:1 dr, and 95% ee. Maleimido-substituted dimethyl ester cyclopropane 2b was successfully reacted, affording annulation adduct 3n in good results. Replacing the succinimide group with phthalimide increased reactivity but decreased enantioselectivity ( 3a vs 3o ). With thyminyl-substituted D-A aminocyclopropane 2d as the reactant, the [3 + 2] annulation could proceed under Cu(OTf) 2 - L4 as the catalyst, affording chiral thymine carbocyclic nucleoside analog 3p in 81% yield, 1.9:1 dr, and 67% ee. The absolute configuration of 3a was assigned by X-ray diffraction analysis. The relative configuration of diastereomer 3o′ was also assigned by X-ray crystallography. Fig. 3: Substrate scope of the reaction. Unless otherwise noted, reaction conditions are as follows: Ni(OTf) 2 / L4 (1:1.2, 5 mol%), 1 (0.2 mmol), 2 (0.44 mmol) in CH 2 Cl 2 (4.0 mL) at 25 °C under N 2 for 24 h. Isolated total yields for product 3 (both diastereoisomers) were reported. The dr value was determined by 1 H NMR spectra of the crude product. The ee value was determined by chiral HPLC analysis. a Reaction conditions: 1a (0.3 mmol), 2a (0.66 mmol) in CH 2 Cl 2 (6.0 mL). b Reaction time: 36 h. c Reaction conditions: Cu(OTf) 2 / L4 (1:1.2, 10 mol%) at 50 °C for 64 h. d Reaction temperature: 0 °C. e Reaction conditions: Cu(OTf) 2 / L4 (1:1.2, 10 mol%) at 35 °C. Full size image Kinetic resolution experiment and scale-up reaction In the above [3 + 2] annulation reaction, excess aminocyclopropane (2.2 equiv.) was used, which influenced ee value of 3a . Thus, the kinetic resolution of aminocyclopropane 2a was performed (Fig. 4a ). At 62% conversion, recovered aminocyclopropane 2a was obtained in 87% ee, and product 3a was obtained in 40% yield, 8:1 dr, and 95% ee. Furthermore, a gram-scale synthesis of tricyclic indoline 3a was carried out (Fig. 4b ). Using 5 mol% of Ni(OTf) 2 -PyIPI L4 , 4 mmol of indole 1a reacted smoothly with aminocyclopropane 2a , affording 1.12 g (70% yield) of product 3a with 11:1 dr and 96% ee. After recrystallization, indoline 3a was obtained as a pure enantiomer (63% yield, 99% ee). Fig. 4: Kinetic resolution experiment and scale-up reaction. a Kinetic resolution experiment of 3-methylindole 1a with aminocyclopropane 2a . b Gram-scale synthesis of tricyclic indoline 3a . Full size image Mechanistic studies To understand the mechanism of the reaction catalyzed by Ni(OTf) 2 -PyIPI L4 , a series of control experiments were performed (Fig. 5 ). Firstly, ligand L10 , the N -Me derivative of L4 , was evaluated, generating product 3a in low yield (45%) and reduced enantioselectivity (67% ee). This indicated that N‒H proton on the imidazolidine moiety was crucial for enhanced reactivity and enantioselectivity. In the case of ligand L11 , bearing a phenyl ring instead of pyridine ring, only trace amount of product 3a was obtained. By eliminating the pyrroloimidazolone moiety (ligand L12 ), once again only trace amount of product 3a was obtained. When ligands L13 and L14 , lacking imidazolidine moieties, were examined, the yields and enantioselectivities were poor. Therefore, according to the obtained data the tridentate nitrogen coordinated to Ni(II) ion was essential for reactivity and stereocontrol. Fig. 5: Control experiments. Reaction conditions: Ni(OTf) 2 / L (1:1.2, 5 mol%), 1a (0.1 mmol), 2a (0.22 mmol) in CH 2 Cl 2 (2.0 mL) at 25 °C under N 2 for 24 h; The total yield ( 3a + 4a ) and dr value of 3a were determined by 1 H NMR spectra of the crude product; The ee value of 3a was determined by chiral HPLC analysis. Full size image Examination of the relationship between the enantioselectivity of ligand L4 and product 3a (Fig. 6 ) revealed a linear correlation in the catalytic reaction, which indicated that the species, 1:1 ratio of L4 to Ni(II), may be the active catalytic species for the reaction. Fig. 6: Mechanism investigation. The relationship between ee values of ligand L4 and product 3a . Full size image The Ni(OTf) 2 -PyIPI L4 -catalyzed reaction mechanism and stereoselectivity were extensively examined by using density functional theory (DFT). Firstly, the structure of complex c-2a was studied in detail by theoretical calculations and X-ray crystallography, which were displayed in Supplementary Figs. 131 – 132 . As described in Fig. 7 , the mechanism consisted of a two-step process: ring-opening and ring-closing. In step 1, Ni(OTf) 2 -PyIPI L4 and ( S )-aminocyclopropane 2a generated complex c - 2a , in which pentacoordinated Ni(II) formed square pyramidal geometry due to the steric repulsion of a phenyl group in the imidazolidine moiety of L4 . PyIPI L4 acted as a tridentate ligand with three nitrogen atoms coordinated to Ni(II) and ( S )- 2a as a bidentate substrate with two carbonyl oxygen atoms coordinated to Ni(II). Meanwhile, the imidazolidine NH of L4 formed H-bond with the oxygen atom in succinimide moiety, and π–π stacking interaction was observed between two aryl groups in the imidazolidine moiety. Then, the reactant complex ( RC ) was formed from indole 1a and complex c - 2a , followed by ring-opening of indole 1a to ( S )- 2a from the indole’s Si face via transition state TS1 with the relative free energy of 20.7 kcal/mol. Intermediate IM1 formed the C3-alkylation indole zwitterion. Fig. 7: Catalytic reaction pathway. Relative energy profiles (in kcal/mol) of catalyzed reaction pathway and optimized structures of important transition state (bond lengths, Å) at the M06-2X-D3/Def2-TZVP/SMD(DCM)//M06-2X-D3/Def2-SVP level. Full size image In step 2, intermediate IM2 was generated via bond rotation from IM1 , which allowed restoration of H-bond between the imidazolidine NH of L4 and the oxygen atom in succinimide moiety. The ring-closing at C2 position of the indole proceeded via transition state TS2 with the relative free energy of 26.0 kcal/mol, affording complex PC1 . Addition of substrate 2a released tricyclic indoline 3a and complex c - 2a was regenerated. Based on the energetic span model [39] of catalytic cycles, the reaction rate was determined by TS2 (26.0 kcal/mol) and IM1 (−3.0 kcal/mol). Furthermore, as shown in Supplementary Fig. 133 , there was a bifurcating transition state [40] TS3 between TS1 and IM1 in the reaction pathways. 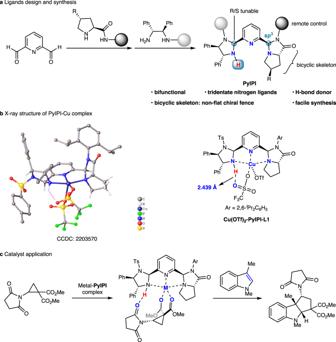Fig. 2: Design, synthesis, and application of PyIPI ligands. aDesign and synthesis of PyIPI ligands.bX-ray structure of Cu(OTf)2-PyIPIL1complex.cMetal-PyIPI complex catalyzed asymmetric dearomative [3 + 2] annulation of indoles with donor–acceptor aminocyclopropane. PyIPI imidazoline-pyrroloimidazolone pyridine. Meanwhile, the other pathway would lead to intermediate IM3 which corresponded to product 4a . This phenomenon corresponeded to 1,2-alkyl group migration [41] , [42] , [43] in the experimental study. Interestingly, from the viewpoint of the activation energy barrier, the side-pathway was energetically more favored than the main-pathway. However, from another perspective, in the dynamic competition between IM1 and IM3 , the nucleophilic attack of N lone pair at the nearby C2 atom in indole 1a to form a double bond would lead to the dominant IM1 intermediate. Importantly, the relative free energy of IM1 was 6.4 kcal/mol lower than that of IM3 , and was even 3.0 kcal/mol lower than reactant, which indicated that IM1 was the high fraction stable intermediate. Thus, C3-alkylation product 3a was the main product and was consistent with the above experiments (Table 1 , entry 18). The stereoselectivity of the [3 + 2] annulation reaction was further explored by comparing the geometry information and free energy of the enantio-determining transition states (Fig. 8 ). As mentioned above, the ring-closing step was the rate-determining step. The relative free energy of TS2 was 2.4 kcal/mol (ΔΔ G ‡ ) lower than that of ent -TS2 , which suggested that (1 R ,3a R ,8b R )- 3a was the dominant adduct, and was in good agreement with the above experiments (Table 1 , entry 18). The visual analysis of non-covalent interactions (NCI) [44] for ent -TS2 was performed by independent gradient model based on Hirshfeld partition (IGMH) [45] , [46] . As shown in the lower right corner of Fig. 8 , it indicated that the observed increase of the energy barrier was mainly caused by the obvious steric repulsion between the indoline ring and phenyl group of the imidazoline moiety. In addition, H-bond interaction between imidazolidine NH and oxygen atom in succinimide moiety in TS2 (2.036 Å) was stronger than that of ent -TS2 (2.894 Å), which was also favorable for lowering the energy barrier in Fig. 8 . Fig. 8: Stereocontrol mechanism. DFT-optimized structures (bond lengths, Å) and relative free energies (∆ G , kcal/mol) of enantio-determining transition states at the M06-2X-D3/Def2-TZVP/SMD(DCM)//M06-2X-D3/Def2-SVP level of theory. Full size image The catalytic asymmetric dearomative [3 + 2] annulation of 3-substituted indoles with D-A aminocyclopropanes is realized. C 1 -Symmetric bifunctional tridentate PyIPI ligand was rationally designed and facilely synthesized with structurally tunable. With 5 mol% of Ni(OTf) 2 -PyIPI L4 complex as the catalyst, diverse tricyclic indolines were obtained in moderate to good yields, good chemoselectivities, high diastereoselectivities (up to 10:1 dr), and excellent enantioselectivities (up to 98% ee). To our surprise, PyIPI L4 with an unusual cis -configuration was the optimal ligand, which was found to be better than C 2 -symmetric tridentate nitrogen ligands L8 and L9 in the annulation reaction. A series of control experiments, as well as single crystal structure of PyIPI L1 -Cu(OTf) 2 complex, linear correlation experiment, and DFT calculations, revealed a dual activation mechanism, where the tridentate nitrogen atoms coordinated with Ni(II) to activate aminocyclopropane via bidentate coordination with the geminal diester, followed by imidazolidine NH formed a H-bond with the oxygen atom in succinimide moiety. In addition, high enantioselectivity of the reaction was governed by steric factors. Further applications of chiral PyIPI in other metal-catalyzed asymmetric reactions are currently underway in our research group. Typical procedure for the synthesis of PyIPI ligand Pyridine-2,6-dicarbaldehyde (20.0 mmol) and L -prolinamides (10.0 mmol) were added to a pressure-resistant test tube with anhydrous ethanol (30.0 mL). Then, the reaction was heated and stirred at 60 °C for 3 h. After that, the reaction mixture was concentrated in vacuo to remove ethanol. The residue was purified by flash column chromatography (Pet/EtOAc, 10/1-1/1, v/v) to give the one-sided condensation product. Then, in a round-bottomed flask containing a stir bar, the above one-sided condensation product (1.0 mmol), ( R , R )-diphenylethylenediamine (1.0 mmol), CH 3 CO 2 H (1.5 mmol, 74.0 μL), and dichloromethane (6.0 mL) were added. Then, the reaction was stirred at 30 °C under N 2 for 6–8 h. After that, the reaction mixture was quenched by aqueous NaHCO 3 . The organic layer was extracted with dichloromethane for 3 times, and the collected organic layer was dried over Na 2 SO 4 . After removing the solvent under reduced pressure, the resulting residue was purified by silica gel column chromatography to give the corresponding PyIPI ligand. 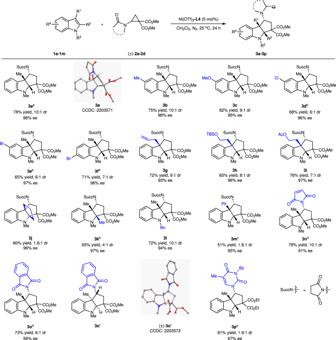Fig. 3: Substrate scope of the reaction. Unless otherwise noted, reaction conditions are as follows: Ni(OTf)2/L4(1:1.2, 5 mol%),1(0.2 mmol),2(0.44 mmol) in CH2Cl2(4.0 mL) at 25 °C under N2for 24 h. Isolated total yields for product3(both diastereoisomers) were reported. The dr value was determined by1H NMR spectra of the crude product. The ee value was determined by chiral HPLC analysis.aReaction conditions:1a(0.3 mmol),2a(0.66 mmol) in CH2Cl2(6.0 mL).bReaction time: 36 h.cReaction conditions: Cu(OTf)2/L4(1:1.2, 10 mol%) at 50 °C for 64 h.dReaction temperature: 0 °C.eReaction conditions: Cu(OTf)2/L4(1:1.2, 10 mol%) at 35 °C. Typical procedure for the catalytic asymmetric dearomative [3 + 2] annulation In a dry reaction tube, a mixture of Ni(OTf) 2 (3.6 mg, 0.01 mmol, 5 mol%), ligand L4 (7.9 mg, 0.012 mmol, 6 mol%), and aminocyclopropane 2 (0.44 mmol) in DCM (3.0 mL) were stirred at room temperature for 30 minutes under the atmosphere of nitrogen. 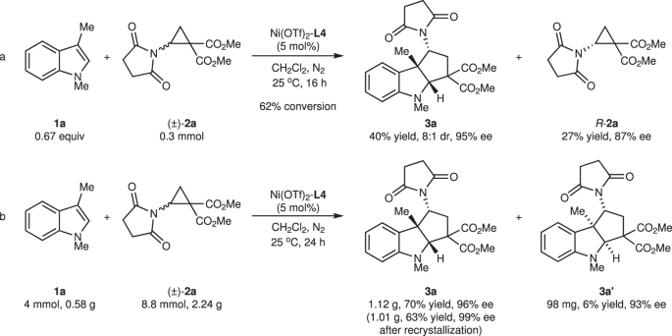Fig. 4: Kinetic resolution experiment and scale-up reaction. aKinetic resolution experiment of 3-methylindole1awith aminocyclopropane2a.bGram-scale synthesis of tricyclic indoline3a. 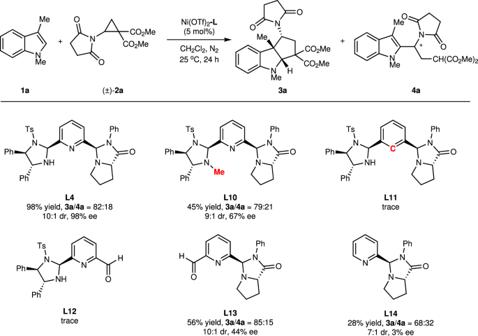Fig. 5: Control experiments. Reaction conditions: Ni(OTf)2/L(1:1.2, 5 mol%),1a(0.1 mmol),2a(0.22 mmol) in CH2Cl2(2.0 mL) at 25 °C under N2for 24 h; The total yield (3a+4a) and dr value of3awere determined by1H NMR spectra of the crude product; The ee value of3awas determined by chiral HPLC analysis. Then indole substrate 1 (0.2 mmol) in DCM (1.0 mL) was added to the mixture of catalyst via a syringe. After 24 h, the reaction was complete (monitored by TLC). 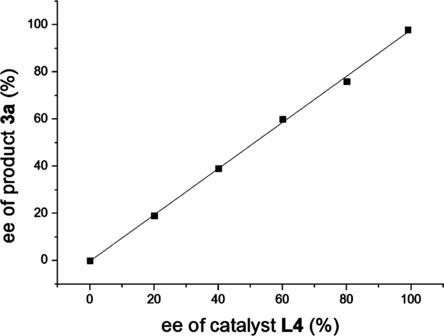Fig. 6: Mechanism investigation. The relationship between ee values of ligandL4and product3a. 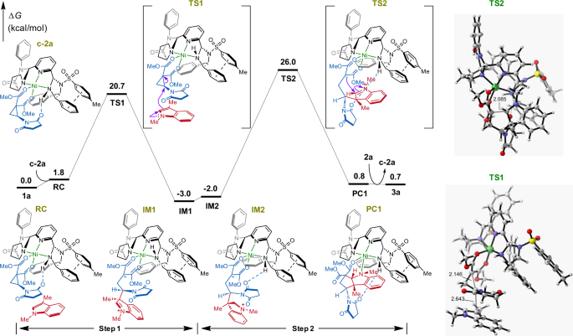Fig. 7: Catalytic reaction pathway. Relative energy profiles (in kcal/mol) of catalyzed reaction pathway and optimized structures of important transition state (bond lengths, Å) at the M06-2X-D3/Def2-TZVP/SMD(DCM)//M06-2X-D3/Def2-SVP level. 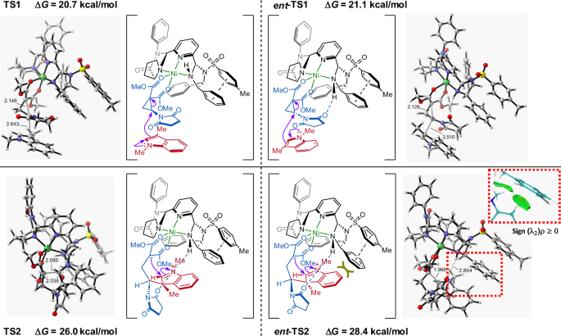Fig. 8: Stereocontrol mechanism. DFT-optimized structures (bond lengths, Å) and relative free energies (∆G, kcal/mol) of enantio-determining transition states at the M06-2X-D3/Def2-TZVP/SMD(DCM)//M06-2X-D3/Def2-SVP level of theory. The reaction was filtered through a glass funnel within layer of silica gel (100–200 mesh) and purified by flash column chromatography (Pet/EtOAc, v/v, 10:1-2:1) to give the product 3 .